Observation of an evolving magnetic flux rope before and during a solar eruption Explosive energy release is a common phenomenon occurring in magnetized plasma systems ranging from laboratories, Earth's magnetosphere, the solar corona and astrophysical environments. Its physical explanation is usually attributed to magnetic reconnection in a thin current sheet. Here we report the important role of magnetic flux rope structure, a volumetric current channel, in producing explosive events. The flux rope is observed as a hot channel before and during a solar eruption from the Atmospheric Imaging Assembly telescope on board the Solar Dynamic Observatory. It initially appears as a twisted and writhed sigmoidal structure with a temperature as high as 10 MK, and then transforms toward a semi-circular shape during a slow-rise phase, which is followed by fast acceleration and onset of a flare. The observations suggest that the instability of the magnetic flux rope triggers the eruption, thus making a major addition to the traditional magnetic-reconnection paradigm. In contrast to a thin current sheet structure, a magnetic flux rope is a volumetric current channel with helical magnetic field lines wrapping around its centre axial field. Both structures can store a large amount of free magnetic energy in the current-carrying magnetic fields. Although it is generally believed that magnetic reconnection occurring in the current sheet releases magnetic energy producing various explosive phenomena [1] , [2] , [3] , [4] , [5] , the role of magnetic flux ropes in the explosive process is less studied and not well understood. Nevertheless, there is recently an increasing interest in flux ropes, especially when a realistic three-dimensional (3D) setting is considered. Laboratory experiments show that two parallel flux ropes can drive magnetic reconnection through magnetohydrodynamic attraction [6] . Large scale 3D numerical simulations have demonstrated that the magnetic reconnection layer is dominated by the formation and interaction of flux ropes [7] . It has been suggested that the observed episodic ejection of plasma blobs in many black hole systems is caused by the formation and ejection of flux ropes [8] . In the research area of solar and heliospheric physics, the magnetic flux rope is considered to be a fundamental structure underlying the phenomenon of coronal mass ejections (CMEs), a well-known driver of space weather that may affect critical technological systems in space and on the ground. The first direct observational evidence of the presence of an isolated magnetic flux rope in the Sun–Earth system is from the near-Earth in situ solar wind observations of the so-called magnetic clouds [9] , [10] . Improved coronagraphic observations of CMEs from the Solar and Heliospheric Observatory showed that CMEs in the outer corona often contain a circular intensity pattern, suggesting the presence of a magnetic flux rope [11] . However, the detection of magnetic flux ropes in the lower corona before the CME formation has been elusive. In fact, one outstanding controversial issue in solar physics, both observationally and theoretically, has been when, where and how the magnetic flux rope is formed. The phenomenon of solar filaments has been interpreted as being due to magnetic flux ropes [12] , [13] , as well as the sigmoidal structures (either forward or reverse S-shaped) often seen in soft X-ray coronal images [14] , [15] , [16] . The origin of a pre-existing flux rope has been suggested to come directly from sub-photosphere emerging into the corona [17] , or alternatively from a sheared arcade in the corona through a flux-cancellation process [18] . However, other observers argue that the sigmoid geometry is of sheared field lines, instead of a flux rope, before an eruption [19] . In the sheared-arcade scenario, numerical simulations show that the magnetic reconnection in the corona could transform the sheared arcade into a flux rope [20] . Here we report on unambiguous observational evidence of the presence of a flux rope before and during a solar eruption on 2011 March 8. The observation was made by the Atmospheric Imaging Assembly (AIA) telescope [21] on board the Solar Dynamic Observatory. The AIA's unprecedented temporal cadence of 12 s, coupled with multi-temperature coronal extreme ultraviolet passbands, enables for the first time the clear observations of the detailed evolution of eruptive structures in the lower corona [22] , [23] , [24] , [25] . The flux rope initially appears as a twisted and writhed sigmoidal structure with a temperature as high as 10 MK. This hot channel then transforms toward a semi-circular shape during a slow rise phase. This phase is followed by the fast acceleration of the hot channel and the onset of an accompanying flare. These observations suggest that the macroscopic instability of the flux rope triggers the eruption, thus making a major addition to the traditional magnetic reconnection paradigm. Hot channel The eruption originated from NOAA Active Region 11171 located at the heliographic coordinates ∼ S21E72. The solar eruption produced an M1.5 class soft X-ray flare on Geostationary Operational Environment Satellite (GOES) scale and a CME with a terminal speed of ∼ 700 km s −1 . The structural evolution of the eruption is shown in Fig. 1 and Supplementary Movies 1 and 2 . The earliest signature of the hot channel started to appear at ∼ 03:31 UT (Universal Time), about 6 min before the onset of the flare. The hot channel only appeared in the AIA's two hottest coronal passbands ( ∼ 10 MK at 131 Å and ∼ 6.4 MK at 94 Å), but is completely absent in the cooler passbands ( ∼ 1.6 MK at 193 Å and ∼ 0.6 MK at 171 Å). The hot channel showed an interesting morphological evolution as it transformed itself from a sigmoidal shape ( Fig. 1d,e ) to a loop-like shape ( Fig. 1f ). The initial sigmoid had a twisted or writhed axis, with its two elbows close to the footpoints extending into the corona and the centre part dipping toward the surface. The dipped centre part then rose up becoming more linear. The continuing rise of the centre part eventually turned the channel into a loop-like shape, or partial torus. During this transformation process, the two footpoints of the evolving hot channel remained fixed. 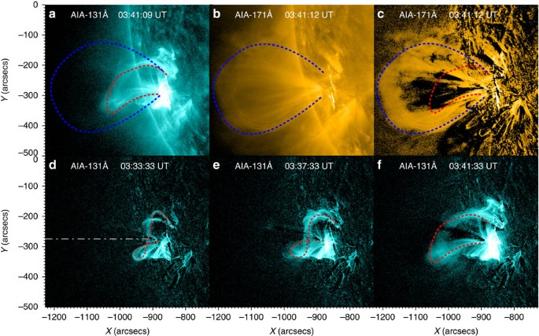Figure 1: Magnetic flux rope seen as a hot channel in Solar Dynamic Observatory/AIA images. The images show three features of the solar eruption on 2011 March 8: a hot channel (indicated by red dotted lines), a cool compression front (indicated by blue dotted lines) and a dark cavity. The time when the image was taken is shown at the top of each panel. (a) Hot coronal image (131 Å,∼10 MK) showing the hot channel at 03:41:09 UT. (b) Cool coronal image (171 Å,∼0.6 MK) at nearly the same time showing the complete absence of the hot channel. (c) The difference coronal image (171 Å, image at 03:41:12 UT, subtracting the base image at 03:20:41 UT) clearly showing the compression front of the eruption. It also shows a dark cavity (the centre dark region in the image) forming inside the enveloping compression front. (d–f) A sequence of base-difference images (131 Å, base image at 03:20:09 UT) showing the evolution of the hot channel. The hot channel apparently transformed from a writhed sigmoidal shape into a semi-circular shape. The white dot-dashed line in panel (d) indicates the position of a slice at which a slice-time plot is constructed to illustrate the full evolution of the eruption features. The full AIA image sequences of the eruption in all six coronal passbands are provided inSupplementary Movies 1and2. Figure 1: Magnetic flux rope seen as a hot channel in Solar Dynamic Observatory/AIA images. The images show three features of the solar eruption on 2011 March 8: a hot channel (indicated by red dotted lines), a cool compression front (indicated by blue dotted lines) and a dark cavity. The time when the image was taken is shown at the top of each panel. ( a ) Hot coronal image (131 Å, ∼ 10 MK) showing the hot channel at 03:41:09 UT. ( b ) Cool coronal image (171 Å, ∼ 0.6 MK) at nearly the same time showing the complete absence of the hot channel. ( c ) The difference coronal image (171 Å, image at 03:41:12 UT, subtracting the base image at 03:20:41 UT) clearly showing the compression front of the eruption. It also shows a dark cavity (the centre dark region in the image) forming inside the enveloping compression front. ( d – f ) A sequence of base-difference images (131 Å, base image at 03:20:09 UT) showing the evolution of the hot channel. The hot channel apparently transformed from a writhed sigmoidal shape into a semi-circular shape. The white dot-dashed line in panel ( d ) indicates the position of a slice at which a slice-time plot is constructed to illustrate the full evolution of the eruption features. The full AIA image sequences of the eruption in all six coronal passbands are provided in Supplementary Movies 1 and 2 . Full size image We also carried out a kinematic analysis of the hot channel ( Figs 2 and 3 ). The entire eruption process as seen by AIA can be divided into two distinct phases: a slow-rise phase before the flare onset and a fast acceleration phase after the flare onset. The slow-rise phase lasted for about 6 min from ∼ 03:31 to 03:37 UT. The hot channel started to appear in the beginning of this phase and then slowly and steadily rose up with an average velocity of ∼ 60 km s −1 ; at the end of this phase, the velocity increased to about ∼ 100 km s −1 . This slow-rise phase was then followed by a much more energetic phase that was accompanied by multiple explosive signatures, including the fast acceleration of the hot channel, the formation of a cool compression front running ahead of the hot channel, the growth of a dark cavity, and a flare of electromagnetic radiation. It has been known that the onset of the fast acceleration phase of CMEs coincides well with the onset of accompanying flares [26] . However, the high cadence observations for this event show that the difference of the two onset times may be as small as 1 min (as indicated by the vertical line on the right in Figs 2 and 3 ). During the fast acceleration phase, the velocity of the hot channel increased from 100 to 700 km s −1 , with an average acceleration about ∼ 1600 m s −2 , which is at least ten times stronger than that in the slow-rise phase. 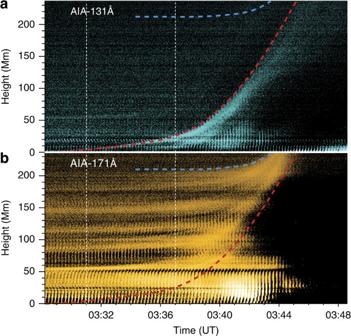Figure 2: Time evolution of the hot channel and compression front. The constructed slice-time plots illustrate the rising motion of the eruption on 2011 March 8. (a) Slice-time plot of AIA 131 Å images showing the rise motion of the hot channel. (b) Slice-time plot of 171 Å images showing the rising motion of the cool compression front. The positions of the hot channel and the compression front are outlined by the red and blue dashed lines, respectively. The white vertical dashed line on the left indicates the start time of the slow-rise phase of the hot channel. The white vertical dashed line on the right indicates the onset time of the accompanying solar flare; this same line also marks the onset of the fast acceleration phase of the hot channel. Figure 2: Time evolution of the hot channel and compression front. The constructed slice-time plots illustrate the rising motion of the eruption on 2011 March 8. ( a ) Slice-time plot of AIA 131 Å images showing the rise motion of the hot channel. ( b ) Slice-time plot of 171 Å images showing the rising motion of the cool compression front. The positions of the hot channel and the compression front are outlined by the red and blue dashed lines, respectively. The white vertical dashed line on the left indicates the start time of the slow-rise phase of the hot channel. The white vertical dashed line on the right indicates the onset time of the accompanying solar flare; this same line also marks the onset of the fast acceleration phase of the hot channel. 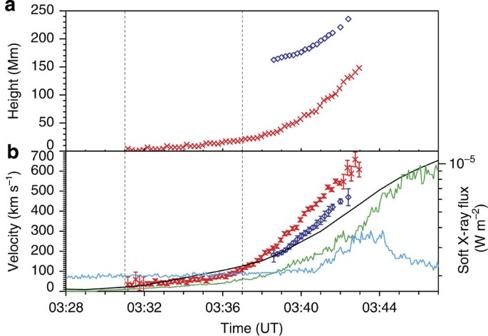Figure 3: Kinematic evolution of eruption features on 2011 March 8. (a) The height–time plots of the hot channel (red cross symbols) and the compression front (blue diamond symbols). The uncertainty of the height measurement is about 2 Mm, whose error bar size is much smaller than the symbol sizes. (b) The velocity–time plots of the hot channel (red cross symbols) and the compression front (blue diamond symbols). The velocity uncertainty is about 30 km s−1. The error bar size is similar to the symbol size. The flux profiles of the accompanying flare are overlaid on the velocity plots: GOES soft X-ray 1–8 Å (black line), RHESSI (Reuven Ramaty High Energy Solar Spectroscopic Imager) hard X-ray 6–12 keV (green line) and 25–50 keV (cyan line). The vertical dashed line on the left indicates the start time of the slow-rise phase of the hot channel. The vertical dashed line on the right indicates the onset time of the accompanying solar flare; this same line also marks the onset of the fast acceleration phase of the hot channel. Full size image Figure 3: Kinematic evolution of eruption features on 2011 March 8. ( a ) The height–time plots of the hot channel (red cross symbols) and the compression front (blue diamond symbols). The uncertainty of the height measurement is about 2 Mm, whose error bar size is much smaller than the symbol sizes. ( b ) The velocity–time plots of the hot channel (red cross symbols) and the compression front (blue diamond symbols). The velocity uncertainty is about 30 km s −1 . The error bar size is similar to the symbol size. The flux profiles of the accompanying flare are overlaid on the velocity plots: GOES soft X-ray 1–8 Å (black line), RHESSI (Reuven Ramaty High Energy Solar Spectroscopic Imager) hard X-ray 6–12 keV (green line) and 25–50 keV (cyan line). The vertical dashed line on the left indicates the start time of the slow-rise phase of the hot channel. The vertical dashed line on the right indicates the onset time of the accompanying solar flare; this same line also marks the onset of the fast acceleration phase of the hot channel. Full size image The bright but cool front of the eruption, best seen in AIA 171 Å ( Figs 1c and 2b ), is believed to be a compression front. It was apparently caused by the compression of the plasma surrounding the hot channel. The compression front only formed late in the fast acceleration phase. The magnetic structure of the active region presumably had two components: one internal core region composed of a flux rope, and one external enveloping region consisting of near-potential magnetic fields. The expansion of the envelope fields formed the bright front through compression. The expansion also explains the development of a dark cavity behind the compression front, as best seen in Fig. 1c , because of the rarefaction of the volume. The velocity of the compression front is always smaller than that of the hot channel throughout the fast acceleration phase ( Fig. 3b ), indicating that the eruption is mainly driven by the hot channel. Flux rope We conclude that the observed evolving hot channel is a magnetic flux rope. It is the coherent helical magnetic field lines that maintain the structure of the channel during the violent eruption process, even though its centre axis changes from a twisted sigmoidal shape to a semi-circular shape, and even though the structure undergoes an acceleration as strong as almost six times the solar surface gravitational acceleration (274 m s −2 ). The two ends of the flux rope remain anchored onto the photosphere, because of the line-tying effect. The observed morphological evolution resembles the result of the 3D numerical simulation of a magnetic flux rope [16] . We further conclude that the magnetic flux rope has fully formed before the onset of the eruption. The onset of the eruption is clearly marked by the onset of the flare and the fast acceleration of the flux rope. The initial sigmoidal-shaped flux rope formed even before the slow-rise phase. Therefore, the flux rope should have formed during the period of the relative quiescent evolution of the source active region, which can last for days or weeks. It could also form through an interior dynamo process before its emergence to the surface. The observational result described above has serious theoretical implications. It makes a major addition to the standard paradigm of eruptive flares, the so-called CSHKP model [27] , [28] , [29] , [30] . The CSHKP model and its many variants assume that the current-sheet magnetic configuration is of primary importance; the magnetic reconnection in the current sheet releases the magnetic energy that produces flare emission, flare ribbons and post-flare loop arcades. Nevertheless, the standard model does not explicitly address the trigger of the eruption. Our work provides strong evidence that the trigger is the instability of a pre-existing flux rope. The reconnecting current sheet is likely formed underneath the rising flux rope through the upward stretching of surrounding magnetic fields. One such mechanism of triggering is the so-called torus instability [31] , [32] , an ideal magnetohydrodynamic process responsible for the loss of equilibrium of a toroidal current ring. In the torus instability model, a critical vertical gradient of the external magnetic field determines the instability. The appearance of the instability should mark the separation between the slow-rise phase and the fast acceleration phase, corresponding to the onset of the eruption. The fast-rising motion of the flux rope may create a current sheet underneath and drive plasma inflow toward the current sheet, resulting in fast magnetic reconnection. In this scenario, the occurrence of fast magnetic reconnection is not spontaneous; instead, it is driven by the macroscopic motion of a magnetic flux rope. Our result suggests magnetic flux ropes have an important role in triggering and driving the explosive energy release process in solar eruptions, and possibly in many other plasma systems in space and laboratories. Data and observations The AIA instrument on the Solar Dynamic Observatory provides the essential observations of the flux rope. The AIA instrument has ten passbands, six of which are sensitive to coronal temperatures mainly contributed from emissions of specific spectral lines. The six coronal passbands, in the order of decreasing temperature, are 131 Å (Fe XXI, ∼ 10 MK), 94 Å (Fe XVIII, ∼ 6.4 MK), 335 Å (Fe XVI, ∼ 2.5 MK), 211 Å (Fe XIV, ∼ 2.0 MK), 193 Å (Fe XII, ∼ 1.6 MK), and 171 Å (Fe IX, ∼ 0.6 MK), respectively. Each AIA image has 4096×4096 pixels (0.6″ pixel size, 1.5″ spatial resolution) covering the full disk of the Sun and up to 0.5 R ⊙ above the limb. The observational cadence of the AIA is one image every 12 s at each passband. The AIA images shown in this paper ( Fig. 1 and Supplementary Movies 1 and 2 ) are a small portion of the original full size images. The X-ray data of the flare, as shown in Fig. 3 , are from two instruments. The soft X-ray data are from the GOES that provides the integrated full-disk soft X-ray emission from the Sun. The GOES soft X-ray data have been historically used to characterize the magnitude, onset time and peak time of solar flares. The hard X-ray data are from the Reuven Ramaty High Energy Solar Spectroscopic Imager spacecraft. Kinematic analysis The kinematic information of the hot channel and the compression front, as shown in Fig. 3 , is obtained by analysing AIA images. We visually inspect the images and identify the leading edges of these features. The heights are measured from the projected distance of the leading edges from the initial position of the hot channel. The measurement of the hot channel is made on AIA 131 Å images, whereas that of the compression front is on AIA 171 Å images. The uncertainty of the height measurement is about four pixels, or 2 Mm, which is much smaller than the size of the height symbols used in Fig. 3 . On the basis of the height–time measurements, the velocities are then derived from the numerical derivative method that uses Lagrangian interpolation of three neighbouring points. To reduce the uncertainty of the derived velocities, the height points are smoothed using a cubic spline interpolation method. The derived velocity uncertainty is about 30 km s −1 . As shown in Fig. 3 , the velocity error bars are about the same size as the symbols, except for the edge points. How to cite this article: Zhang, J. et al . Observation of an evolving magnetic flux rope before and during a solar eruption. Nat. Commun. 3:747 doi: 10.1038/ncomms1753 (2012).